HIV-1 Rev downregulates Tat expression and viral replication via modulation of NAD(P)H:quinine oxidoreductase 1 (NQO1) HIV-1 gene expression and replication largely depend on the regulatory proteins Tat and Rev, but it is unclear how the intracellular levels of these viral proteins are regulated after infection. Here we report that HIV-1 Rev causes specific degradation of cytoplasmic Tat, which results in inhibition of HIV-1 replication. The nuclear export signal (NES) region of Rev is crucial for this activity but is not involved in direct interactions with Tat. Rev reduces the levels of ubiquitinated forms of Tat, which have previously been reported to be important for its transcriptional properties. Tat is stabilized in the presence of NAD(P)H:quinine oxidoreductase 1 (NQO1), and potent degradation of Tat is induced by dicoumarol, an NQO1 inhibitor. Furthermore, Rev causes specific reduction in the levels of endogenous NQO1. Thus, we propose that Rev is able to induce degradation of Tat indirectly by downregulating NQO1 levels. Our findings have implications in HIV-1 gene expression and latency. HIV-1 encodes two regulatory proteins, Tat and Rev. Tat is known to interact with the TAR ( trans -activating responsive) element [1] and increase the steady-state levels of all the viral transcripts. Rev, on the other hand, is mainly involved in the transport of singly spliced or unspliced HIV-1 genomic RNA via a cis -acting element called Rev response element [2] , [3] , [4] and downregulates the levels of Tat, Rev and Nef messenger RNA (mRNAs) [5] The cytoplasmic transport of Rev response element-containing mRNAs encoding structural proteins results in a switch from early Rev-independent to Rev-dependent gene expression associated with late stages of the viral life cycle. The regulatory feedback mechanisms governed by Tat and Rev ensure the delicate balance between early and late infection. Tat and Rev proteins are able to shuttle between the nucleus and cytoplasm and potentially perform functions in both of these cellular compartments [6] , [7] , [8] , [9] . Both Tat and Rev extensively exploit various cellular factors to govern viral gene expression [10] , [11] . The regulatory and accessory proteins of HIV-1 enhance viral replication and govern pathogenesis by interacting with many cellular proteins and hijacking cellular machinery for promoting its own replication by overcoming various host restriction factors [12] . HIV-1 proteins also interact with one another to modulate various functions; Vif is reported to degrade the Vpr protein and Nef promotes the degradation of Tat [13] , [14] , [15] . Controlled degradation of cellular proteins is necessary for normal metabolism of the cell [16] . Proteasomal and lysosomal degradation are two major cellular pathways for protein degradation [17] . The ubiquitin–proteasomal pathway is the major pathway for the degradation of proteins [18] ; however, many proteins with intrinsically unfolded structures are degraded in an ubiquitin-independent manner using the 20S proteasomal pathway [19] , [20] . The free 20S proteasome present in the cell degrades proteins that have unstructured domains, including proteins that are in their oxidized states [20] , [21] . The 20S proteasomal degradation is a widespread phenomenon; since more than 30% of total cellular proteins possess substantial intrinsic structural disorders, they may be undergoing 20S proteasome-mediated degradation [19] , [22] . 20S proteasomal degradation is a passive process that only needs unstructured regions in the substrate protein [20] .This pathway is reported to promote the degradation of many key cellular proteins such as p53, p73, p21, PGC1-α, BIMEL and so on that possess unstructured regions [23] , [24] , [25] , [26] . The process is primarily controlled by NADH-bound NAD(P)H:quinine oxidoreductase 1(NQO1), which associates with 20S proteasome and inhibits this pathway [20] , [27] . The competitive removal of NADH from NQO1 with chemical compounds such as dicoumarol {3,3′-methylenebis(4-hydroxy-2H-chromen-2-one}, curcumin and diminutol activates this pathway by enhancing the degradation of unstructured proteins [20] , [23] , [25] , [27] . While extensive work has been carried out in finding out about host proteins interacting with regulatory and/or structural proteins of HIV-1, relatively little work has been carried out to address the functional implications of viral protein–protein interactions. It was earlier shown that Tat and Vpr [13] or Tat and Nef [15] interact with each other with significant functional consequences with respect to gene expression. This prompted us to ask whether Tat can interact with other regulatory and accessory proteins of HIV-1. As, HIV-1 Tat and Rev are two important regulatory proteins of virus, we set out to investigate whether Rev may influence the levels of Tat and vice versa. Here we show that the levels of Tat are specifically reduced in presence of Rev, which results in decrease of HIV-1 gene expression and replication significantly. We observed that NQO1 stabilizes Tat protein in a dose-dependent manner and the inhibitor of NQO1, dicoumarol, potently induces degradation of the Tat protein and inhibits HIV-1 replication. On the other hand, Rev downmodulates the expression of NQO1 in a dose-dependent manner. These observations have very significant implications with respect to controlling HIV-1 gene expression and latency. Rev reduces activity of Tat by inducing its degradation The effect of Rev on Tat-mediated HIV-1 LTR-promoter activation was investigated by three independent experiments. The genes encoding Myc-Tat and Myc-Rev were expressed in HEK-293T cells along with HIV-1 LTR-luciferase or the reporter HIV-1 provirus (pNL4-3-luciferase). A Rev-dose-dependent inhibition of Tat-mediated reporter gene activation was observed ( Fig. 1a , 1st panel). A robust reduction in the expression of pNL4-3-luciferase was also observed ( Fig. 1a , 2nd panel). Similarly, Rev also caused a potent inhibition of HIV-1 gene expression/replication in the presence of exogenous Tat ( Fig. 1a , 3rd panel). We next explored the effect of Rev on the expression of Tat by co-expressing them in HEK-293T (Human embryonic kidney-293T cells) and CHME3 cells (human microglial cells, natural target of HIV-1 infection) [28] , which showed almost complete reduction in Tat levels ( Fig. 1b,c , left panels). We also measured Tat protein level in HEK-293T cells co-transfected with Flag-Tat HIV-1 DNA (in pNL4.3 back bone), and Myc-Rev. CHME3 cells were also infected with vesicular stomatitis virus envelope G glycoprotein (VSV-G)-pseudotyped pNL4.3-Flag-Tat virus (MOI 0.5) along with Myc-Rev. Tat protein was significantly reduced by Rev and significant inhibition of viral gene expression (as detected by p24 antigen by western blotting) was observed in both HEK-293T and CHME3 cells ( Fig. 1b,c , right panels). HIV-1 subtype-C Rev also caused significant decrease in levels of Tat ( Supplementary Fig. 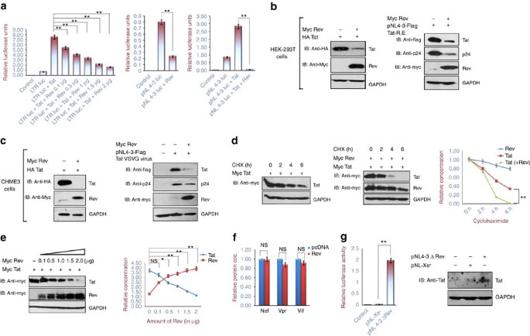Figure 1: Rev decreases Tat-mediated HIV-1 LTR promoter activation and viral replication by degrading Tat. (a) HEK-293T cells were co-transfected with LTR-Luc, renilla luciferase (normalization control), pCMV-Myc-Tat and increasing dose of pCMV-Myc-Rev, or with pNL4-3-Luc, Renilla luciferase and pCMV-Myc-Rev or with pCMV-Myc-Rev, pCMV-Myc-Tat and pNL4.3-Luc followed by measurement of luciferase activity. The graphs were plotted after normalizing the reading with the renilla luciferase reading. (b) HEK-293T cells were transfected with pCMV-HA-Tat or pNL4.3. Flag-Tat along with Rev followed by western blotting (WB) of Tat and Rev. (c) CHME3 cells were either transfected with pCMV-HA-Tat and pCMV-Myc-Rev, or transfected with pCMV-Myc-Rev and infected with VSV-G-psuedotyped pNL4-3-Flag-Tat virus followed by WB. (d) HEK-293T cells were transfected either with pCMV-Myc-Tat alone or with pCMV-Myc-Rev; 36 h post transfection, CHX was added to stop protein synthesis and cells were harvested at different time periods followed by WB of Tat and Rev. Protein levels of Tat and Rev were plotted against CHX treatment period. (e) A fixed dose of Tat plasmid was transfected along with increasing dose of Rev to study the dose-dependent effect of Rev on the Tat protein level. WB was done after a period of 24 h of transfection to measure the level of Tat and Rev proteins in the cell lysates. Densitometry was done using ImageJ software. (f) The levels of HIV-1 Nef, Vpr and Vif in the presence of Rev were measured by transfecting pCMV-Myc-Nef, pCMV-Myc-Vpr and pCMV-Myc-Vif along with pCMV-Myc-Rev in HEK-293T cells. WB image was quantified using imageJ software and plotted. (g) TZM-bl cells were transfected with pNL-Xe−and pNL4-3ΔRev as indicated, followed by the luciferase assay. Tat was also blotted using anti-Tat antiserum. Data obtained are represented as mean±s.e.m. of three independent experiments.Pvalue was calculated by a two-tailedt-test (*P<0.05, **P<0.01; NS, not significant). Full blots are shown inSupplementary Fig. 13. 1 ) Figure 1: Rev decreases Tat-mediated HIV-1 LTR promoter activation and viral replication by degrading Tat. ( a ) HEK-293T cells were co-transfected with LTR-Luc, renilla luciferase (normalization control), pCMV-Myc-Tat and increasing dose of pCMV-Myc-Rev, or with pNL4-3-Luc, Renilla luciferase and pCMV-Myc-Rev or with pCMV-Myc-Rev, pCMV-Myc-Tat and pNL4.3-Luc followed by measurement of luciferase activity. The graphs were plotted after normalizing the reading with the renilla luciferase reading. ( b ) HEK-293T cells were transfected with pCMV-HA-Tat or pNL4.3. Flag-Tat along with Rev followed by western blotting (WB) of Tat and Rev. ( c ) CHME3 cells were either transfected with pCMV-HA-Tat and pCMV-Myc-Rev, or transfected with pCMV-Myc-Rev and infected with VSV-G-psuedotyped pNL4-3-Flag-Tat virus followed by WB. ( d ) HEK-293T cells were transfected either with pCMV-Myc-Tat alone or with pCMV-Myc-Rev; 36 h post transfection, CHX was added to stop protein synthesis and cells were harvested at different time periods followed by WB of Tat and Rev. Protein levels of Tat and Rev were plotted against CHX treatment period. ( e ) A fixed dose of Tat plasmid was transfected along with increasing dose of Rev to study the dose-dependent effect of Rev on the Tat protein level. WB was done after a period of 24 h of transfection to measure the level of Tat and Rev proteins in the cell lysates. Densitometry was done using ImageJ software. ( f ) The levels of HIV-1 Nef, Vpr and Vif in the presence of Rev were measured by transfecting pCMV-Myc-Nef, pCMV-Myc-Vpr and pCMV-Myc-Vif along with pCMV-Myc-Rev in HEK-293T cells. WB image was quantified using imageJ software and plotted. ( g ) TZM-bl cells were transfected with pNL-Xe − and pNL4-3ΔRev as indicated, followed by the luciferase assay. Tat was also blotted using anti-Tat antiserum. Data obtained are represented as mean±s.e.m. of three independent experiments. P value was calculated by a two-tailed t -test (* P <0.05, ** P <0.01; NS, not significant). Full blots are shown in Supplementary Fig. 13 . Full size image The effect of Rev on the half-life of Tat was studied by cycloheximide (CHX) chase assay. After 6 h of chase, >50% reduction was observed in the intracellular levels of Tat ( Fig. 1d , 1st and 3rd panels), but only ∼ 10% reduction in Rev ( Supplementary Fig. 2 ). The CHX chase experiment showed almost complete disappearance of Tat after 4 h of chase in presence of Rev ( Fig. 1d , 2nd and 3rd panels). The degradation of Tat was observed as soon as it was expressed ( Supplementary Fig. 3 ). Thus, we conclude that half-life of Rev is significantly more than that of Tat, and Rev decreases the half-life of Tat very potently. A progressive decrease in the expression of Tat was observed with increasing amounts of Rev ( Fig. 1e ). The same was confirmed with the red fluorescent protein-tagged Tat construct ( Supplementary Fig. 4 ). The levels of Nef, Vpr and Vif were unaffected by Rev ( Fig. 1f ; Supplementary Fig. 5 ), indicating the specificity of Rev-mediated degradation of Tat. TZM-bl cells were also transfected with pNL-Xe − (envelope mutated) and pNL4-3ΔRev as indicated in Fig. 1g . LTR-luciferase activity was found to be higher with pNL4-3ΔRev ( Fig. 1g , 1st panel). The expression of Tat was also found to be higher in pNL4-3ΔRev ( Fig. 1g , 2nd panel). All the above results led us to conclude that Rev specifically downregulates the expression of Tat in a dose-dependent manner. Rev induces proteasomal degradation of Tat Next, we examined the mechanism of Rev-mediated Tat degradation by measuring Tat mRNA level using real-time PCR (RT-PCR) or blocking cellular proteasome by MG132 treatment and measuring Tat protein level in presence or absence of Rev in HEK-293T cells. To check the effect of Rev on transcription of the Tat gene, quantitative (q)RT-PCR analysis was performed ( Fig. 2a ). The mRNA level of Tat remained almost unaffected ( Fig. 2a , 1st panel), whereas the intracellular levels of Tat protein in the same fraction showed a significant reduction in the presence of Rev ( Fig. 2a , 2nd panel). The level of Tat protein was largely restored in the presence of MG132 ( Fig. 2b , 1st panel). Similar results were obtained with pNL4-3-Flag-Tat ( Fig. 2b , 2nd panel). These data support the involvement of proteasomal machinery in Rev-mediated degradation of Tat. Proteins are ubiquitinated before being targeted to proteasome-mediated degradation. However, an earlier report showed that ubiquitination of Tat is important for its transcriptional activity [29] . We, therefore, tested the effect of Rev on ubiquitinated Tat as described earlier [30] . Rev potently reduced the ubiquitinated forms of Tat ( Fig. 2c ), which may explain the reduced functional activity of Tat shown earlier. The above results suggest that Rev induces proteasomal degradation of Tat protein in a ubiquitin-independent manner. To further rule out the involvement of ubiquitination in the process of Rev-mediated Tat protein degradation, the ubiquitination was inhibited by a dominant-negative ubiquitin mutant (HA-UbKO) having all seven lysine residues mutated with arginine [31] . As shown in Fig. 2d , the expression of Tat protein was not restored to original levels in HA-UbKO-transfected cells. This was further confirmed by treating the cells with PYR-41 (50 μM), a specific inhibitor of ubiquitin-activating enzyme E1 (ref. 32 ), thereby inhibiting whole-cell ubiquitination ( Supplementary Fig. 6 ), and the effect of Rev on Tat was observed. PYR-41 treatment of cells failed to restore the levels of Tat protein ( Fig. 2e ), as both PYR-41 untreated and -treated cells showed a ∼ 50% reduction in expression of Tat by Rev confirming that Tat degradation by Rev does not involve ubiquitination machinery. 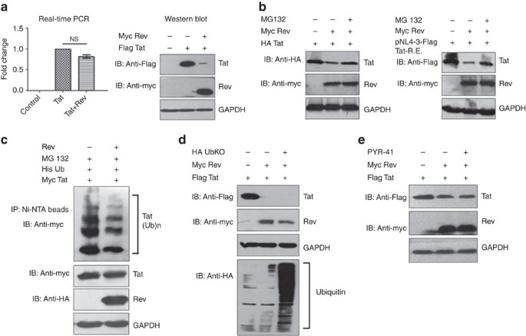Figure 2: Rev-mediated downregulation of Tat is a post-translational effect. (a) HEK-293T cells were transfected with pcDNA3.1-Tat-Flag alone or with pCMV-Myc-Rev, after 24 h cells were harvested and divided into two equal parts. One half was used for real-time qPCR as described in Methods. Mean values and s.d. were calculated from 2dCtof three independent experiments and plotted.Pvalues were calculated by a two-tailedt-test (NS, not significant).The other half was analysed by western blotting using specific antibodies. (b) HEK-293T cells were transfected with pcDNA3.1-Tat-HA alone or with pCMV-Myc-Rev; after 24 h the cells were treated with 20 μM MG132 for 8 h followed by western blotting. Similarly, pNL4-3-Flag-Tat-R.E. was transfected alone or with pCMV-Myc-Rev followed by MG132 (20 μM) treatment for 8 h and immunoblotted for Flag-Tat. (c) HEK-293T cells were transfected with 6 × His–Ub, pCMV-Myc-Tat alone or with pCMV-HA-Rev, incubated for 24 h and treated with 20 μM MG132 for 8 h before harvesting. Ubiquitinated proteins were purified under denaturing condition with Ni-NTA beads as described in Methods and analysed by western blotting. Ubiquitinated Tat protein was probed using anti-Myc antibody. (d) HEK-293T cells were transfected with pcDNA3.1-Flag-Tat, pCMV-Myc-Rev and HA-Ub KO; after 24 h incubation, cell lysate was prepared and the proteins were analysed by western blotting. (e) HEK-293T cells were transfected with pcDNA3.1-Flag-Tat and pCMV-Myc-Rev for 24 h followed by treatment with PYR-41 (50 μM) for 6 h as indicated, and proteins were analysed by western blotting. Full blots are shown inSupplementary Fig. 14. Figure 2: Rev-mediated downregulation of Tat is a post-translational effect. ( a ) HEK-293T cells were transfected with pcDNA3.1-Tat-Flag alone or with pCMV-Myc-Rev, after 24 h cells were harvested and divided into two equal parts. One half was used for real-time qPCR as described in Methods. Mean values and s.d. were calculated from 2 dCt of three independent experiments and plotted. P values were calculated by a two-tailed t -test (NS, not significant).The other half was analysed by western blotting using specific antibodies. ( b ) HEK-293T cells were transfected with pcDNA3.1-Tat-HA alone or with pCMV-Myc-Rev; after 24 h the cells were treated with 20 μM MG132 for 8 h followed by western blotting. Similarly, pNL4-3-Flag-Tat-R.E. was transfected alone or with pCMV-Myc-Rev followed by MG132 (20 μM) treatment for 8 h and immunoblotted for Flag-Tat. ( c ) HEK-293T cells were transfected with 6 × His–Ub, pCMV-Myc-Tat alone or with pCMV-HA-Rev, incubated for 24 h and treated with 20 μM MG132 for 8 h before harvesting. Ubiquitinated proteins were purified under denaturing condition with Ni-NTA beads as described in Methods and analysed by western blotting. Ubiquitinated Tat protein was probed using anti-Myc antibody. ( d ) HEK-293T cells were transfected with pcDNA3.1-Flag-Tat, pCMV-Myc-Rev and HA-Ub KO; after 24 h incubation, cell lysate was prepared and the proteins were analysed by western blotting. ( e ) HEK-293T cells were transfected with pcDNA3.1-Flag-Tat and pCMV-Myc-Rev for 24 h followed by treatment with PYR-41 (50 μM) for 6 h as indicated, and proteins were analysed by western blotting. Full blots are shown in Supplementary Fig. 14 . Full size image Rev NES is important for Tat downregulation To determine the domains of Rev involved in degradation of Tat, ΔNLS (nuclear localization signal)-Mt and ΔNES-Mt of Rev were generated by mutagenesis as described earlier [33] and confirmed by sequencing ( Fig. 3a ), and their effect on the expression of Tat was investigated. As expected, Rev-Wt caused almost complete degradation of Tat; ΔNLS-Mt also caused a similar effect, but the ΔNES-Mt failed to exhibit degradation ( Fig. 3b ). HIV-1 replication was also tested in the presence of the same mutants of Rev. As expected, pNL4-3-luc showed significant luciferase activity, which was severely reduced in the presence of Rev-Wt and RevΔNLS-Mt but not in the presence of RevΔNES-Mt ( Fig. 3c ). Further to test whether nuclear export signal (NES) alone can induce the degradation of Tat, a 12-aa-long NES peptide (LQLPPLERLTLD) was fused with glutathione S -transferase (GST) and co-transfected with haemagglutinin (HA)-Tat in HEK-293T cells. GST-NES failed to induce the degradation of Tat ( Fig. 3d ). This suggested that the NES peptide alone was not sufficient to cause degradation of Tat and that the other regions of the Rev protein may also be involved in this process. 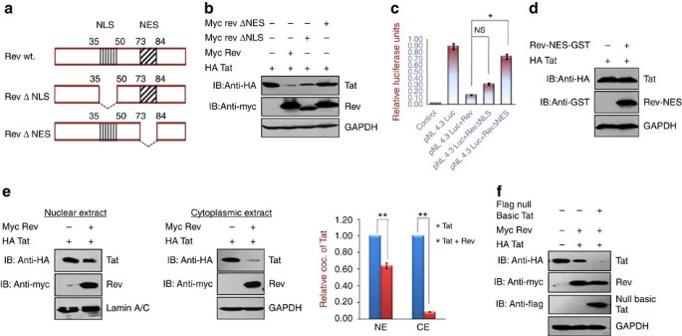Figure 3: Deletion of the NES region of Rev abrogates Tat degradation, indicating that this phenomenon occurs in the cytoplasm. (a) NLS (35-50aa) and NES (73–84) regions of Rev were deleted to make RevΔNLS and RevΔNES mutant constructs, respectively. (b) Tat-expressing plasmid (pcDNA3.1-Tat-HA) was transfected alone or with pCMV-Myc-Rev or pCMV-Myc-RevΔNLS or pCMV-Myc-RevΔNES in HEK-293T cells and the level of Tat protein was measured by western blotting. (c) Effect of Rev mutants on HIV-1 replication was observed by the transfection of pNL4-3-luc along with pCMV-Myc-Rev, pCMV-Myc-RevΔNLS and pCMV-Myc-RevΔNES in HEK-293T cells, followed by the luciferase assay. (d) Effect of the NES region of Rev on Tat stability was measured by transfecting pcDNA3.1-Tat-HA and pGST-NES in HEK-293T cells, followed by western blotting for Tat protein. (e) HEK-293T cells were transfected with pcDNA3.1-Tat-HA and pCMV-Myc-Rev, the nuclear and cytoplasmic extracts were prepared separately followed by western blotting for Tat and Rev proteins. The relative band intensity of Tat and Rev proteins were measured by ImageJ and plotted. (f) CHME3 cells were transfected with pcDNA3.1-Tat-HA, pCMV-Myc-Rev and pcDNA3.1-Flag-NB-Tat (Nullbasic-Tat mutant) and the Tat protein level was analysed by western blotting. Data obtained are represented as mean±s.e.m. of three independent experiments.Pvalue was calculated by a two-tailedt-test (*P<0.05, **P<0.01; NS, not significant). Full blots are shown inSupplementary Fig. 15. Figure 3: Deletion of the NES region of Rev abrogates Tat degradation, indicating that this phenomenon occurs in the cytoplasm. ( a ) NLS (35-50aa) and NES (73–84) regions of Rev were deleted to make RevΔNLS and RevΔNES mutant constructs, respectively. ( b ) Tat-expressing plasmid (pcDNA3.1-Tat-HA) was transfected alone or with pCMV-Myc-Rev or pCMV-Myc-RevΔNLS or pCMV-Myc-RevΔNES in HEK-293T cells and the level of Tat protein was measured by western blotting. ( c ) Effect of Rev mutants on HIV-1 replication was observed by the transfection of pNL4-3-luc along with pCMV-Myc-Rev, pCMV-Myc-RevΔNLS and pCMV-Myc-RevΔNES in HEK-293T cells, followed by the luciferase assay. ( d ) Effect of the NES region of Rev on Tat stability was measured by transfecting pcDNA3.1-Tat-HA and pGST-NES in HEK-293T cells, followed by western blotting for Tat protein. ( e ) HEK-293T cells were transfected with pcDNA3.1-Tat-HA and pCMV-Myc-Rev, the nuclear and cytoplasmic extracts were prepared separately followed by western blotting for Tat and Rev proteins. The relative band intensity of Tat and Rev proteins were measured by ImageJ and plotted. ( f ) CHME3 cells were transfected with pcDNA3.1-Tat-HA, pCMV-Myc-Rev and pcDNA3.1-Flag-NB-Tat (Nullbasic-Tat mutant) and the Tat protein level was analysed by western blotting. Data obtained are represented as mean±s.e.m. of three independent experiments. P value was calculated by a two-tailed t -test (* P <0.05, ** P <0.01; NS, not significant). Full blots are shown in Supplementary Fig. 15 . Full size image Rev-mediated degradation of Tat is predominant in cytoplasm NES region of Rev facilitates the transport of protein from nucleus to cytoplasm of cell and its deletion causes the accumulation of protein in the nucleus. Since NES peptide alone was unable to cause degradation ( Fig. 3d ) and deletion of the NES region of Rev inhibited the Tat degradation ( Fig. 3b ), we reasoned that degradation of Tat might be occurring in cytoplasm. To check this possibility, the nuclear (NE) and cytoplasmic (CE) extracts were analysed separately for degradation of Tat. Tat degradation was predominantly observed in CEs, as there is ∼ 90% reduction in CE compared with ∼ 40% reduction in NE ( Fig. 3e ). This was further confirmed in HIV-1-susceptible CHME3 cells using the Flag-Null-basic Tat construct (NB-Tat), which is known to induce the accumulation of Rev in the cytoplasm [34] . When NB-Tat was co-expressed with Tat and Rev in CHME3 cells, degradation of Tat was enhanced ( Fig. 3f ) suggesting that Rev-mediated degradation of Tat occurs primarily in the cytoplasmic compartment of the cell. Deletion of the NLS region of Rev inhibits Tat–Rev interaction To explore whether Tat interacts with Rev directly, co-immunoprecipitation was carried out with lysates prepared from HA-Rev- and Myc-Tat-transfected HEK-293T cells using anti-HA antibody-conjugated beads. Myc-Tat gets pulled down in HA-Rev-transfected cells but not in Rev-untransfected cells ( Fig. 4a ). To probe the direct interaction between Tat and Rev, the yeast two-hybrid assay was performed, which showed that Tat directly interacts with Rev ( Supplementary Fig. 7 ). To explore the effect of NLS and NES deletion mutants of Rev on Tat–Rev interaction, they were overexpressed in HEK-293T cells and immunoprecipitation was carried out. Rev-Wt and ΔNES-Mt showed interaction with Tat, but deletion of the NLS region abrogated this interaction ( Fig. 4b ). Since deletion of the NLS region of Rev did not affect degradation of Tat but inhibited its interaction with Tat and NES mutant of Rev showed interaction with Tat (which does not degrade Tat), we concluded that Rev-mediated Tat degradation is independent of Tat–Rev interaction and some cellular protein/proteins may be mediating this process. This observation prompted us to explore other pathways by which Tat may be degraded. 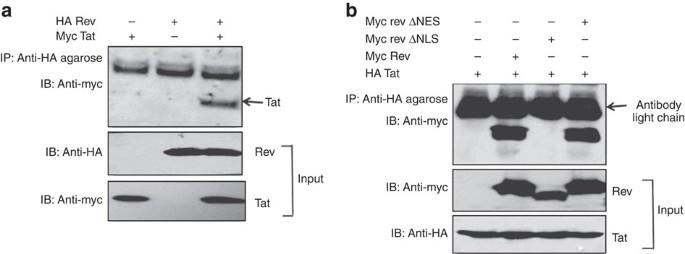Figure 4: HIV-1 Tat and Rev interact with each other and deletion of the NLS region of Rev abrogates the interaction. (a) HEK-293T cells were transfected with pCMV-HA-Rev and pCMV-Myc-Tat as indicated. Cell extracts were subjected to immunoprecipitation using anti-HA antibody-conjugated protein A agarose beads as described in Methods, followed by western blotting using the anti-myc antibody. (b) HEK-293T cells were transfected with HA-Tat, pCMV-Myc-Rev, pCMV-Myc-RevΔNLS and pCMV-Myc-RevΔNES. Cell extracts were subjected to immunoprecipitation using anti-HA antibody-conjugated protein A agarose beads followed by western blotting using anti-myc antibody. Full blots are shown inSupplementary Fig. 15. Figure 4: HIV-1 Tat and Rev interact with each other and deletion of the NLS region of Rev abrogates the interaction. ( a ) HEK-293T cells were transfected with pCMV-HA-Rev and pCMV-Myc-Tat as indicated. Cell extracts were subjected to immunoprecipitation using anti-HA antibody-conjugated protein A agarose beads as described in Methods, followed by western blotting using the anti-myc antibody. ( b ) HEK-293T cells were transfected with HA-Tat, pCMV-Myc-Rev, pCMV-Myc-RevΔNLS and pCMV-Myc-RevΔNES. Cell extracts were subjected to immunoprecipitation using anti-HA antibody-conjugated protein A agarose beads followed by western blotting using anti-myc antibody. Full blots are shown in Supplementary Fig. 15 . Full size image Dicoumarol degrades Tat and inhibits HIV-1 replication Multiple functions of Tat are governed by its disorderness, which enables it to interact with multiple cellular proteins [35] . We verified the unstructured nature of Tat protein using multiple algorithms. These programs predicted different degrees of intrinsic disorderness in the Tat protein. The fold index program showed complete disorderness in Tat protein along its entire length with no folded regions ( Supplementary Fig. 8a ). Other programs such as RONN, metaPrDOS and FoldUnfold also predicted substantial unfolded regions in the Tat protein ( Supplementary Fig. 8b–d ). The intrinsically disordered proteins are prone to degradation through 20S proteasome [19] , [20] . To investigate whether HIV-1 Tat is degraded through the 20S proteasomal pathway, Myc-Tat-transfected cells were treated with dicoumarol. After 4 h of 200 μM dicoumarol treatment, Tat protein levels decreased by >50% and at 400 μM dicoumarol concentration Tat levels decreased by >90%, showing a dose-dependent decrease of Tat with dicoumarol ( Fig. 5a ). The treatment of dicoumarol did not affect the levels of Vpr, Nef and Gag (p55) (which are comparatively more structured) proteins both at 200- and 400-μM doses ( Supplementary Fig. 9 ). The time needed for dicoumarol-induced Tat degradation was also investigated using a fixed dose (400 μM) of dicoumarol. There was a progressive decrease in the levels of Tat protein with 3–6 h of treatment, and after 12 h, a complete degradation of Tat was observed ( Fig. 5b ). Since dicoumarol induces degradation of intrinsically unfolded proteins, so its treatment should enhance the rate of degradation of Tat protein that can be measured by the CHX chase assay. Treatment of CHX reduced the levels of Tat protein in a time-dependent manner; however, simultaneous treatment with dicoumarol further increases the rate of Tat reduction ( Fig. 5c ). 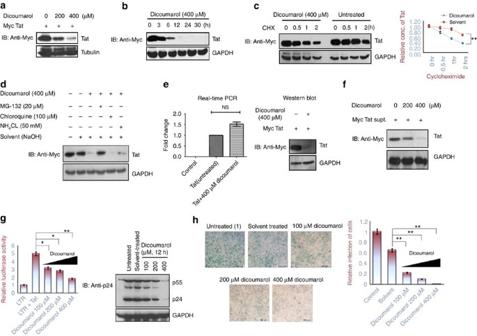Figure 5: Dicoumarol induces HIV-1 Tat protein degradation and inhibits HIV-1 LTR transactivation and viral replication. (a–c) HEK-293T cells were transfected with pCMV-Myc-Tat and treated with dicoumarol and/or cycloheximide as indicated and immunoblotting for Tat was done; the band intensity of Tat was measured and plotted against treatment time. (d) HEK-293T cells were transfected with pCMV-Myc-Tat and incubated for 24 h, subsequently the cells were treated with dicoumarol alone or with MG132, chloroquine, ammonium chloride as indicated for 6 h, followed by western blotting (WB). (e) HEK-293T cells were transfected with pCMV-Myc-Tat and treated with dicoumarol for 6 h, cells were harvested and equally divided into two parts. One half was used for total RNA isolation followed by real-time qPCR using Tat-specific primers. Mean values and s.d. were calculated from 2dCtof three independent experiments and plotted.Pvalues were calculated by a two-tailedt-test (*P<0.05, **P<0.01; NS, not significant). Second half was subjected to immunoblotting for Tat. (f) Tat protein-containing cell culture medium from pCMV-Myc-Tat-transfected cells was used to treat HEK-293T cells for 4 h followed by treatment with dicoumarol as described in Methods. Cell lysates were analysed by WB using anti-myc antibody. (g) pCMV-Myc-Tat-transfected TZM-bl cells were treated with dicoumarol for 12 h and the LTR-luciferase assay was performed (first panel). Tumour-necrosis factor-α-stimulated HIV-1-producing J1.1 cells were also treated with dicoumarol followed by WB for p24 protein (second panel). (h) Cell culture medium obtained from dicoumarol-treated J1.1 cells from a previous experiment containing HIV-1 particles was used to infect TZM-bl cells and the infected cells were detected by β-galactosidase staining. Scale bars, 500 μM. Data obtained are represented as mean±s.e.m. of three independent experiments.Pvalue was calculated by a two-tailedt-test (*P<0.05, **P<0.01; NS, not significant). Full blots are shown inSupplementary Fig. 16. Figure 5: Dicoumarol induces HIV-1 Tat protein degradation and inhibits HIV-1 LTR transactivation and viral replication. ( a–c ) HEK-293T cells were transfected with pCMV-Myc-Tat and treated with dicoumarol and/or cycloheximide as indicated and immunoblotting for Tat was done; the band intensity of Tat was measured and plotted against treatment time. ( d ) HEK-293T cells were transfected with pCMV-Myc-Tat and incubated for 24 h, subsequently the cells were treated with dicoumarol alone or with MG132, chloroquine, ammonium chloride as indicated for 6 h, followed by western blotting (WB). ( e ) HEK-293T cells were transfected with pCMV-Myc-Tat and treated with dicoumarol for 6 h, cells were harvested and equally divided into two parts. One half was used for total RNA isolation followed by real-time qPCR using Tat-specific primers. Mean values and s.d. were calculated from 2 dCt of three independent experiments and plotted. P values were calculated by a two-tailed t -test (* P <0.05, ** P <0.01; NS, not significant). Second half was subjected to immunoblotting for Tat. ( f ) Tat protein-containing cell culture medium from pCMV-Myc-Tat-transfected cells was used to treat HEK-293T cells for 4 h followed by treatment with dicoumarol as described in Methods. Cell lysates were analysed by WB using anti-myc antibody. ( g ) pCMV-Myc-Tat-transfected TZM-bl cells were treated with dicoumarol for 12 h and the LTR-luciferase assay was performed (first panel). Tumour-necrosis factor-α-stimulated HIV-1-producing J1.1 cells were also treated with dicoumarol followed by WB for p24 protein (second panel). ( h ) Cell culture medium obtained from dicoumarol-treated J1.1 cells from a previous experiment containing HIV-1 particles was used to infect TZM-bl cells and the infected cells were detected by β-galactosidase staining. Scale bars, 500 μM. Data obtained are represented as mean±s.e.m. of three independent experiments. P value was calculated by a two-tailed t -test (* P <0.05, ** P <0.01; NS, not significant). Full blots are shown in Supplementary Fig. 16 . Full size image Dicoumarol induces proteasomal degradation of Tat The levels of Tat protein were largely restored upon MG132 treatment, while treatment with lysosomal inhibitors such as chloroquine or ammonium chloride failed to do so ( Fig. 5d ). To rule out any effect of dicoumarol on the Tat gene transcription itself, a real-time qPCR assay was performed. pCMV-Myc-Tat-transfected HEK-293T cells were treated with 400 μM dicoumarol and cells were divided into two parts: one was used for immunoblotting to measure Tat protein level and the other was used to measure Tat mRNA level after isolation of total RNA. Real-time PCR showed that dicoumarol treatment does not reduce Tat mRNA level significantly, whereas the protein level gets reduced significantly as shown by western blot ( Fig. 5e ), confirming that dicoumarol specifically reduces the Tat protein level. To further rule out the effect of dicoumarol on Tat gene transcription, Tat protein present in the cell culture medium of Tat-expressing cells was applied to HEK-293T cells followed by dicoumarol treatment for 4 h. Treatment of dicoumarol results in Tat protein reduction in a dose-dependent manner ( Fig. 5f ), confirming the effect of dicoumarol on Tat protein degradation. Dicoumarol reduces activity of Tat and viral production Since the primary function of Tat is to transactivate HIV-1 LTR promoter [12] , the effect of dicoumarol on Tat-mediated LTR transactivation was also studied in TZM-bl cells as described earlier [36] . Treatment of dicoumarol of Tat-transfected TZM-bl cells exhibited significant decrease in the levels of luciferase activity in a dose-dependent manner ( Fig. 5g , 1st panel). Tat expression in TZM-bl cells resulted in an increase in reporter gene activity by approximately fivefold; however, when these cells were treated with 200 μM dicoumarol, the luciferase activity decreased by ∼ 40% and by ∼ 70% at 400 μM dicoumarol concentration confirming the dose effect on the stability of Tat protein. We then examined the possibility of exploiting the effect of dicoumarol on Tat degradation in the context of HIV-1 replication. Since Tat directly controls HIV-1 replication, its degradation should result in reduction of HIV-1 replication [12] , [37] . The effect of dicoumarol on HIV-1 replication was studied in J1.1 cell line [38] , which is a Jurkat E6.1-derived human T lymphocyte chronically infected with HIV-1 and viral replication increases tremendously upon stimulation with tumour-necrosis factor-α (ref. 39 ). The level of p24 decreased with dicoumarol in a dose-dependent manner and there was almost a complete inhibition of HIV-1 replication at 400 μM dicoumarol concentration ( Fig. 5g , 2nd panel). Further there is also a dose-dependent decrease in the infectivity of the released virus from J1.1 cells in response to dicoumarol treatment ( Fig. 5h ). We conclude that dicoumarol potently inhibits HIV-1 replication. Dicoumarol does not cause cell death To rule out the possibility that the observed inhibitory effect of dicoumarol on Tat could be due to the toxicity or cell death, we measured the viability of the dicoumarol-treated cells by propidium iodide (PI) staining [40] . Fluorescence-activated cell sorting analysis revealed that dicoumarol did not cause any significant changes in the viability of the cells at the concentration of 200 μM dicoumarol. At a 400-μM dose, the proportion of dead cells increased only marginally ( Supplementary Fig. 10a ). The effect of dicoumarol on cellular physiology was also tested. As expected, treatment with 400 μM dicoumarol resulted in complete disappearance of Tat; however, its removal for a period of 3 h results in about 50% restoration of Tat protein levels and after 6 h there was a complete restoration ( Supplementary Fig. 10b , 1st panel). Similarly, dicoumarol treatment to pNL4-3-transfected cells resulted in significant reduction in p24 levels, which was restored to 50% by 6 h and almost 100% after 12 h of the removal of dicoumarol ( Supplementary Fig. 10b , 2nd panel). These results indicate that dicoumarol did not affect the protein-synthesizing machinery adversely. Tat is stabilized by NQO1, inhibitor of 20S proteasome The degradation of Tat by dicoumarol and its subsequent inhibitory effect on HIV-1 replication clearly indicates that the degradation of Tat is accomplished through the 20S proteasomal pathway. However, to further confirm this finding, we studied the effect of NQO1 protein, which is an inhibitor of this proteasomal pathway, on the stability of Tat. NQO1 expression in HEK-293T cells caused an increase in the levels of Tat protein in a dose-dependent manner ( Fig. 6a , 1st panel). NQO1-transfected cells also showed an increased Tat protein level in comparison with untransfected cells when the cells were treated with cell culture medium containing Tat protein ( Fig. 6a , 2nd panel), confirming the stabilization of Tat protein by NQO1. The functional consequences of Tat stabilization in response to NQO1 were also validated by investigating the effect of NQO1 on HIV-1 replication. We observed a dose-dependent increase in viral replication (detected by p24 and p55 levels) in the presence of NQO1 ( Fig. 6b ). To further confirm the role of NQO1 in Tat stabilization, Tat-transfected cells were treated with diminutol, another inhibitor of NQO1 activity, and the level of Tat protein was measured by western blotting. Treatment of 400 μM diminutol for 6 h showed almost a complete degradation of Tat comparable to Tat level in 400-μM dicoumarol-treated cells ( Supplementary Fig. 11 ). 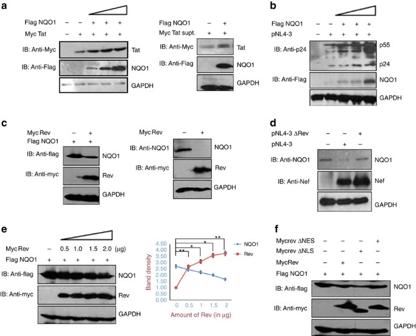Figure 6: NQO1 expression results in the increase of Tat protein level as well as viral replication, whereas Rev downregulates NQO1. (a) HEK-293T cells were co-transfected with pCMV-Myc-Tat and different doses of pcDNA3.1-Flag-NQO1, the cells were incubated for 36 h followed by immunoblotting for Tat and NQO1 (first panel). Also the Tat protein-containing cell culture medium from pCMV-Myc-Tat-transfected cells was used to treat HEK-293T cells expressing pcDNA3.1-Flag-NQO1 as described in Methods. Cell lysates were analysed by WB using anti-myc and anti-Flag antibodies. (b) pNL4-3 was co-transfected with pcDNA3.1-Flag-NQO1 and pNL4-3 in HEK-293T cells and p24 level was measured by immunoblotting. (c) pcDNA3.1-Flag-NQO1 was expressed alone or with pCMV-Myc-Rev in HEK-293T cells followed by western blotting using anti-Flag antibody, and endogenous NQO1 level was measured using anti-NQO1 antibody. (d) HEK-293T cells were transfected with pNL4-3 and pNL4-3ΔRev as indicated and after 24 h of transfection, levels of NQO1 and Nef were measured by western blotting with anti-NQO1 and anti-Nef antibodies, respectively. (e) Increasing dose of pCMV-Myc-Rev was transfected with a fixed dose of pcDNA3.1-Flag-NQO1; immunoblotting for Flag-NQO1 and Myc-Rev was done after 36 h of incubation. Data obtained are represented as mean±s.e.m. of three independent experiments.Pvalue was calculated by a two-tailedt-test (*P<0.05, **P<0.01, not significant). (f) HEK-293T cells were transfected with pcDNA3.1-Flag-NQO1 alone or with pCMV-Myc-Rev or pCMV-Myc-RevΔNLS or pCMV-Myc-RevΔNES and immunoblotted. Full blots are shown inSupplementary Figs 16 and 17. Figure 6: NQO1 expression results in the increase of Tat protein level as well as viral replication, whereas Rev downregulates NQO1. ( a ) HEK-293T cells were co-transfected with pCMV-Myc-Tat and different doses of pcDNA3.1-Flag-NQO1, the cells were incubated for 36 h followed by immunoblotting for Tat and NQO1 (first panel). Also the Tat protein-containing cell culture medium from pCMV-Myc-Tat-transfected cells was used to treat HEK-293T cells expressing pcDNA3.1-Flag-NQO1 as described in Methods. Cell lysates were analysed by WB using anti-myc and anti-Flag antibodies. ( b ) pNL4-3 was co-transfected with pcDNA3.1-Flag-NQO1 and pNL4-3 in HEK-293T cells and p24 level was measured by immunoblotting. ( c ) pcDNA3.1-Flag-NQO1 was expressed alone or with pCMV-Myc-Rev in HEK-293T cells followed by western blotting using anti-Flag antibody, and endogenous NQO1 level was measured using anti-NQO1 antibody. ( d ) HEK-293T cells were transfected with pNL4-3 and pNL4-3ΔRev as indicated and after 24 h of transfection, levels of NQO1 and Nef were measured by western blotting with anti-NQO1 and anti-Nef antibodies, respectively. ( e ) Increasing dose of pCMV-Myc-Rev was transfected with a fixed dose of pcDNA3.1-Flag-NQO1; immunoblotting for Flag-NQO1 and Myc-Rev was done after 36 h of incubation. Data obtained are represented as mean±s.e.m. of three independent experiments. P value was calculated by a two-tailed t -test (* P <0.05, ** P <0.01, not significant). ( f ) HEK-293T cells were transfected with pcDNA3.1-Flag-NQO1 alone or with pCMV-Myc-Rev or pCMV-Myc-RevΔNLS or pCMV-Myc-RevΔNES and immunoblotted. Full blots are shown in Supplementary Figs 16 and 17 . Full size image HIV-1 Rev downregulates the expression of NQO1 Our earlier experiments suggested that both HIV-1 Rev and dicoumarol induced the destabilization of HIV-1 Tat protein, and dicoumarol is a specific inhibitor of NQO1, which caused stabilization of the Tat protein. Hence, we next explored the effect of Rev on the expression of NQO1. Exogenously expressed as well as endogenous NQO1 was potently reduced in the presence of Rev ( Fig. 6c ). We then asked whether Tat could have a similar effect on NQO1 as Rev. In both systems (transfected and endogenous), the levels of NQO1 remained unaltered ( Supplementary Fig. 12 ). Taken together, we concluded that Rev specifically reduces NQO1 levels, while Tat does not show such an effect. To investigate the role of Rev in reducing NQO1 levels in viral context, HEK-293T cells were transfected with either pNL4-3 or pNL4-3ΔRev and endogenous NQO1 levels were measured. Expression of pNL4-3 resulted in decrease of NQO1 level, whereas pNL4-3ΔRev expression showed no effect on it ( Fig. 6d ), confirming that HIV-1 Rev induces the downregulation of NQO1. When NQO1 was overexpressed in the presence of increasing doses of Rev as indicated, reduction in levels of NQO1 was observed ( Fig. 6e ). ΔNLS-Mt was able to reduce NQO1 levels very potently (even better than Rev-Wt), while the ΔNES-Mt of Rev failed to do so ( Fig. 6f ). The significant finding of this work is the remarkable ability of Rev to cause specific degradation of Tat, as other accessory proteins were not affected. Rev alone was sufficient to induce this degradation in the absence of other viral gene products. Tat is by far the single most important protein of HIV-1 for enhancing gene expression and replication of the virus. The levels of Tat have also been implicated in latency. By a series of experiments we show that Rev leads to marked reduction in HIV-1 gene expression, which correlated with the decrease in intracellular levels of Tat. While Rev was earlier reported to modulate the mRNA levels of various HIV-1 transcripts [5] , this is the first report showing post-translational regulation of Tat by Rev involving proteasomal machinery. The decrease in intracellular half-life of Tat in the presence Rev by the CHX chase experiment clearly suggested the role of Rev in the degradation of Tat. The experiment also suggested that intracellular half-life of Rev was significantly longer than Tat, with obvious implications in gene expression and latency. HIV-1 latency arises when the intracellular levels of the regulatory protein Tat falls below a critical threshold level. The Rev-mediated Tat degradation experiments using RevΔNLS and RevΔNES mutants clearly suggested that the NES region of Rev was critically important for this activity, while deletion of the NLS region of Rev did not affect its ability to degrade Tat. The inability of this RevΔNES mutant to degrade Tat also correlated with its failure to inhibit HIV-1 gene expression and replication. NES peptide when fused to GST failed to degrade Tat, which indicates that the NES domain of Rev is not sufficient in inducing Tat degradation. Since the NES region of Rev is responsible for exporting Rev from nucleus, we speculated that Rev-mediated degradation of Tat may be occurring in the cytoplasm. This was confirmed when NE and CE were analysed separately in Rev-mediated Tat degradation experiments. This is why NLS-mutated Rev is more efficient than wild-type Rev. It was earlier reported that transcriptional properties of Tat are positively regulated by ubiquitin [29] . Our experiments clearly showed that Rev reduces ubiquitinated forms of Tat and this could be one potential mechanism for reduction of the functional activities of Tat in response to Rev protein. Since NES mutant of Rev showed interaction with Tat protein (which does not degrade Tat) by a pull-down assay, we speculated that this degradation is Tat–Rev interaction independent and may involve additional cellular components. We, therefore, explored alternative pathways by which Tat protein could be degraded. The intrinsic disorder of Tat protein indicated that it could be a potential substrate of the 20S proteasomal pathway and indeed it was potently degraded by dicoumarol as well as diminutol, the activators of this pathway. Tat was potently degraded by dicoumarol at 400 μM concentration in a short period of time (4–8 h post treatment). This rapid inhibitory effect against HIV-1 Tat protein may result in the long-term suppression of HIV-1 or may significantly delay any escape mutants. The observed decrease in Tat protein level in response to dicoumarol treatment was not due to decrease in the Tat gene transcription or cellular toxicity, because it remained unaffected by dicoumarol treatment. The reduction of Tat protein by dicoumarol in the presence of exogenous Tat clearly rules out any inhibitory role of dicoumarol in Tat gene transcription. Further using the CHX chase assay, we found that the rate of degradation of Tat protein was increased significantly when the Tat-expressing cells were treated with dicoumarol. The observed degradation of Tat in response to dicoumarol treatment occurred through the proteasomal pathway, because MG132 treatment led to the inhibition of dicoumarol-induced degradation of Tat protein. The dicoumarol-mediated degradation of Tat is equally effective at the level of the virus production. Chronically infected J1.1 cells (Jurkat T cells), when treated with dicoumarol, showed a significant decrease in the replication of HIV-1. Thus, dicoumarol could be developed as an anti-HIV-1 drug with desirable pharmacogenics parameters suitable for treatment, because it did not cause any irreversible damage to cells. We have clearly showed that dicoumarol treatment itself at indicated doses do not cause any irreversible deleterious effect to cellular physiology. Homologues with desired biological activities of dicoumarol can be synthesized and tested for more potent anti-HIV-1 activity. Rev induced the decrease in levels of endogenous as well as transfected NQO1 in a dose-dependent manner and deletion of Rev from pNL4-3 backbone abrogated HIV-1-mediated downregulation of NQO1, suggesting that Rev regulates the expression of Tat and viral replication indirectly by modulating the expression of NQO1. Mechanistic insights have to be worked out to gain full understanding of the observation. It is noteworthy that here also the NES region of Rev is critically involved. On the contrary, Tat had no effect on the levels of intracellular NQO1. We believe that our data help explain some of the earlier observations, which showed that ectopic expression of Rev inhibits the HIV-1 gene expression and virus production. This observation of Rev-mediated downregulation of viral replication by inducing the degradation of Tat at post-translational level is significantly different from earlier work where Rev was shown to downmodulate the mRNA species of Tat, Rev and Nef [5] . Although our data help explain some of the earlier observations, it does not explain how critical amounts of Tat are maintained for the virus gene expression and replication. It is noteworthy that both Tat and Rev can shuttle between nucleus and cytoplasm, and it is not fully understood as to how the amounts of these two proteins are governed in the two cellular compartments during virus infection. It is tempting to suggest that the amount of Tat that shuttles back in the nucleus is the residual amount that is left post degradation of Tat in the cytoplasmic compartment. Alternatively, the nuclear Tat may also shuttle back in the cytoplasmic compartment, which is then effectively degraded by Rev. Both of these events can potentially augment the ability of Rev to degrade Tat. In summary, we show that the levels of one very important regulatory protein Tat is regulated by another important regulatory protein of HIV, namely Rev. This is accomplished by Rev-mediated modulation of a host protein NQO1 as depicted in the proposed model ( Fig. 7 ). These data have implications for understanding intricacies of complex regulation of HIV-1 replication and latency. 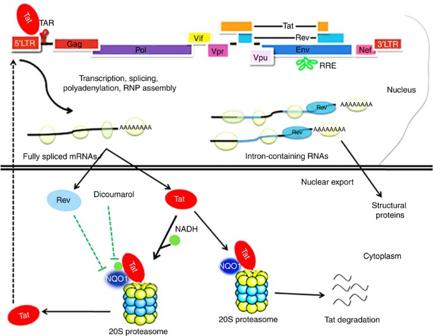Figure 7: Mechanistic model of Rev- and dicoumarol-mediated downregulation of Tat and HIV-1 replication. The initial transcription of HIV-1 genome results in the generation of viral mRNA followed by splicing by host cell machinery to generate fully spliced mRNA encoding Tat, Rev and Nef. These genes are further translated to generate functional proteins. The generation of Tat results in the enhancement of transcription and Rev expression leads to transport of full-length mRNA to the cytoplasm. Rev interacts with the RRE (Rev response element) region present in the viral mRNA and transports it to the cytoplasm for the translation of viral proteins, as well as for packaging of it into the viral particles. The present report demonstrates the degradation of Tat protein through the 20S proteasome. Dicoumarol treatment results in the release of NADH from NQO1 present on the 20S proteasome activating it for the degradation of Tat protein. HIV-1 Rev on the other hand downregulates the NQO1 protein level by enhancing its degradation, which activates the 20S proteasomal pathway resulting in the degradation of Tat protein. The degradation of Tat protein results in the suppression of HIV-1 infectivity through the inhibition of viral replication and virion production. Figure 7: Mechanistic model of Rev- and dicoumarol-mediated downregulation of Tat and HIV-1 replication. The initial transcription of HIV-1 genome results in the generation of viral mRNA followed by splicing by host cell machinery to generate fully spliced mRNA encoding Tat, Rev and Nef. These genes are further translated to generate functional proteins. The generation of Tat results in the enhancement of transcription and Rev expression leads to transport of full-length mRNA to the cytoplasm. Rev interacts with the RRE (Rev response element) region present in the viral mRNA and transports it to the cytoplasm for the translation of viral proteins, as well as for packaging of it into the viral particles. The present report demonstrates the degradation of Tat protein through the 20S proteasome. Dicoumarol treatment results in the release of NADH from NQO1 present on the 20S proteasome activating it for the degradation of Tat protein. HIV-1 Rev on the other hand downregulates the NQO1 protein level by enhancing its degradation, which activates the 20S proteasomal pathway resulting in the degradation of Tat protein. The degradation of Tat protein results in the suppression of HIV-1 infectivity through the inhibition of viral replication and virion production. Full size image Cell culture and transfection HEK-293T (Human embryonic kidney-293T cells), TZM-bl and CHME3 (Human microglial cells) were maintained in DMEM (Himedia Laboratories, India) and J1.1 and E6.1 (Jurkat cells) were cultured in RPMI (Himedia Laboratories) with heat-inactivated 10% fetal bovine serum (Biological Industries) and 100 units penicillin, 0.1 mg streptomycin and 0.25 μg amphotericin B per ml at 37 °C in the presence of 5% CO 2 in a humified incubator. HEK-293T and Jurkat E6.1 cells were purchased from ATCC. TZM-bl and J1.1 were obtained from the NIH AIDS Research Reagent Program, MD, USA. TZM-bl cells contain β-galactosidase and the luciferase gene downstream of HIV-1 LTR promoter [36] . Chronically infected HIV-1-producing cell lines J1.1 were derived from Jurkat E6.1 (ref. 38 ). Transfections were performed using Lipofectamine 2,000 (Invitrogen, USA) and Polyethyleneimine, Linear (MW 25,000; Polysciences Inc., USA) reagents using the manufacturer’s protocol, and the transfection efficiency was always normalized with a reporter gene construct. Plasmids pCMV-Myc-Tat, pCMV-Myc-Rev, pCMV-Myc-Nef, pCMV-Myc-Vpr and pCMV-Myc-Vif plasmids were prepared by cloning pNL4-3-derived genes in pCMV-Myc plasmid from Clontech, USA. Plasmids pCMV-Myc-RevΔNLS and pCMV-Myc-RevΔNES have been described previously [33] . Plasmid pGST-NES is described below in the section ‘NES-specific oligonucleotide cloning’. Renilla luciferase plasmid was a kind gift from Vivek Natrajan, IGIB, Delhi, India. The other plasmids obtained by various sources [31] , [44] , [45] , [46] , [47] , [48] , [49] , [50] , [51] , [52] , [53] , [54] are described in Supplementary Table 1 . Immunoblot analysis HEK-293T cells were transfected with plasmids expressing the gene of interest for 24 h, then the cells were harvested and lysed in RIPA lysis buffer (1% NP-40, 20 mM Tris-HCl, pH 7.5, 150 mM NaCl, 1 mM Na 2 EDTA, 1 mM EGTA, 1% sodium deoxycholate and 1 mM Na 3 VO 4 ). Protein was quantified using the BCA Protein Assay Kit (Pierce, Thermo Scientific, USA). Equal amounts of protein were resolved on SDS–polyacrylamide gel electrophoresis (PAGE) and were transferred to nitrocellulose membrane. The membranes were blocked with 1% BSA and 5% non-fat dry milk (Himedia Laboratories) in 1 × PBS (137 mM NaCl, 2.7 mM KCl, 10 mM Na 2 HPO 4 and 1.8 mM KH 2 PO 4 ) and washed thrice with 1 × PBS containing 0.1% Tween 20 (PBST). Then membranes were incubated with primary antibody, washed with 1 × PBS containing 0.1% Tween 20 and probed with horseradish peroxide (HRP)-conjugated secondary antibody. Blots were developed using ECL (enhanced chemiluminiscent) reagent. Antibodies Anti-c-myc monoclonal antibody (Clontech; 1:1,000), anti-HA-tag polyclonal antibody (Clontech; 1:1,000), anti-GAPDH antibody (Cell Signaling Technology, USA; 1:10,000), anti-Lamin A/C (Cell Signaling Technology; 1:1,000), anti-Flag antibody (Sigma, USA; 1:1,000), anti-His monoclonal antibody (Sigma; 1:1,000), anti-p24 monoclonal antibody (NIH AIDS Reagent Programme, USA; 1:3,000), anti-Nef antibody (NIH AIDS Reagent Programme; 1:2,000), anti-Tat antibody (NIH AIDS Reagent Programme; 1:2,000), anti-NQO1 monoclonal antibody (Santa Cruz Biotechnology, USA; 1:1,000), anti-GST monoclonal antibody (Santa Cruz Biotechnology; 1:1,000), anti-tubulin antibody (Santa Cruz Biotechnology; 1:2,000), anti-rabbit IgG conjugated to HRP (Jackson Immunoresearch, USA; 1:10,000) and anti-Mouse IgG conjugated to HRP (Jackson Immunoresearch; 1:10,000) were used for the western blotting experiments. CHX chase assay To study the degradation kinetics of proteins, the CHX chase assay was performed as described before [30] . HEK-293T cells were transfected with 2 μg each of plasmid DNA for 24 h and then treated with CHX (100 μg ml −1 ; Sigma). Cell lysates were prepared at indicated time points, resolved on 12% SDS–PAGE followed by immunoblotting as described above. Luciferase reporter assay Luciferase reporter assay was performed using the Dual-Luciferase Reporter assay kit (Promega, USA). HEK-293T cells were co-transfected with the luciferase reporter construct and plasmids encoding the desired genes, whereas TZM-bl cells were only transfected with the desired genes. Renilla luciferase construct was used as a control to normalize the transfection efficiency. An empty pcDNA3.1 vector was added to normalize the amount of DNA transfected in each well. At 24 h post transfection, cells were lysed in lysis buffer (Promega). Luciferase activity was measured by a luminometer using two substrates (Promega): one for firefly luciferase and second for renilla luciferase (mixed with stop and glo buffer) with the help of a luminometer (Tecan, Switzerland). The readings of firefly luciferase activity were normalized by renilla luciferase acivity to get true reporter luciferase activity. Real-time PCR RT-qPCR is commonly used to detect RNA expression level in the cell [41] . HEK-293T cells were transfected with the desired plasmid for 24 h, and dicoumarol treatment was done for 6 h where applicable. Total RNA was isolated using Trizol reagent as described by the manufacturer (Invitrogen) and reverse transcribed to form complementary DNA (cDNA) using the cDNA synthesis kit (Promega). One μg of RNA was mixed with random primers and incubated at 70 °C for 15 min and kept at 4 °C. Reverse transcription mix containing 1 × reaction buffer, MgCl2, dNTPs, rRNasin and reverse transcriptase was added to it and incubated at 25 °C for 5 min, 42 °C for 1 h, 70 °C for 15 min and kept at 4 °C. This cDNA was used for SYBR green-based RT-qPCR amplification of the Tat gene using Tat forward primer: 5′-ATGGAGCCAGTAGATCCTAGACTAGAG-3′ and Tat reverse primer: 5′-CGTCGCTGTCTCCGCTTCTTCCT-3′. Human β-actin was used as control and amplified using the primers; forward: 5′-AGGCACCAGGGCGTGAT-3′ and reverse: 5′-GCCCACATAGGAATCCTTCTGAC-3′. Immunoprecipitation The protein–protein interaction was studied by immunoprecipitation. HEK-293T cells were transfected with plasmids encoding the proteins of interest. After 24 h of transfection, cells were harvested and washed with PBS. Cells were lysed in CelLytic M, Cell Lysis Reagent (Sigma) and antibody-conjugated agarose resin (Sigma) was added. It was rotated overnight at 4 °C. After incubation, resin was pelleted and washed with IP buffer (Sigma). It was boiled in 2 × SDS–PAGE loading buffer for 5 min and analysed by western blotting. Yeast two-hybrid assay To analyse the direct interaction between Tat and Rev, they were cloned in pGAD and pGBD plasmids from Clontech. These yeast two-hybrid vectors carry the nutritional markers. The plasmids pGAD and pGBD encode leucine and tryptophan synthesis genes, respectively, which allow yeast cells to grow on minimal media lacking leucine (Leu) or tryptophan (Trp). The yeast two-hybrid assay was performed using reporter yeast strain Saccharomyces cerevisiae AH109 (ref. 42 ). The interaction between Rev and Tat was analysed on SD (synthetic defined; Takara Bio Inc., Japan) plates lacking Leu, Trp and histidine (SD Leu − , Trp − , His − ). Further to investigate the strength of interaction, the transformants were grown on SD plates lacking Leu, Trp, histidine and adenine (SD Leu − , Trp − , His − , Ade − ). In vitro ubiquitination assay In vitro ubiquitination assay was performed to detect ubiquitylated proteins in transfected mammalian cells. HEK-293T cells were co-transfected with a plasmid encoding the desired gene and His–Ub (6 × histidine–ubiquitin) for 24 h and processed as described [30] . Preparation of NEs and CEs This was carried out using NE-PER Nuclear and Cytoplasmic Extraction Reagents (Thermo Scientific). HEK-293T cells were transfected with plasmids of interest and cells were harvested in PBS after 24 h of transfection. Cells were harvested and ice-cold CER I was added to the cell pellet and vortexed vigorously for 15 s to prepare the cell suspension and incubated on ice for 10 min. Ice-cold CER II was then added and vortexed for 5 s and incubated on ice for 1 min. It was again vortexed for 5 s and centrifuged for 5 min at 4 °C. The supernatant was immediately transferred (CE) to a clean pre-chilled tube and stored at −80 °C. The insoluble (pellet) fraction containing nuclei was suspended in ice-cold NER and vortexed for 15 s. It was incubated on ice with vortexing for 15 s every 10 min, for a total of 40 min and centrifuged for 10 min at 4 °C. The supernatant was immediately transferred (NE) to a clean pre-chilled tube and stored at −80 °C. NES-specific oligonucleotide cloning Plasmid pGST-NES was prepared by cloning the following oligonucleotides. Following two short complementary oligonucleotides were synthesized that were specific for the NES region of Rev (1) 5′-GATCCCTTCAGCTACCACCGCTTGAGAGACTTACTCTTGATTAGGC-3′ and (2) 5′-GGCCGCCTAATCAAGAGTAAGTCTCTCAAGCGGTGGTAGCTGAAGG-3′. They were mixed in equal proportion along with 10 × phosphonucleotide kinase buffer, 10 μM ATP, phosphonucleotide kinase enzyme and incubated at 37 °C for 40 min followed by 65 °C for 20 min. NaCl (0.1 M) was added to this mixture and kept for annealing at 94 °C for 4 min, 80 °C for 4 min, 75 °C for 4 min, 70 °C for 10 min, 37 °C for 20 min, 10 °C for 30 min and 4 °C for 2 h. Phosphorylated annealed oligos were diluted and ligated to pEBG vector (Addgene) at BamHI and NotI cloning sites. Dicoumarol treatment Dicoumarol stock solution (70 mM) was made in 0.13 M sodium hydroxide. The stock was diluted in complete medium (DMEM with 10% FCS or RPMI with 10% FCS) to obtain the required concentration and added to the cells. Equal amount of solvent (sodium hydroxide) was added to untreated cells and dicoumarol-treated cells. The cells were harvested after indicated periods of treatment, lysed and probed with specific antibodies. To study the effect of dicoumarol on HIV-1 replication and release from J1.1 cells, tumour-necrosis factor-α-stimulated J1.1 cells were treated with dicoumarol as indicated and supernatant containing virions was collected. The virus-containing medium was used to infect the TZM-bl cells and the infectivity was measured by β-galactosidase staining. The virus-producing J1.1 cells were lysed and probed for p24 antigen by immunoblotting as a measure of virus replication. Sub G o /G 1 DNA content analysis The percentage of cells undergoing apoptosis by dicoumarol treatment was investigated by analysing the sub G o population of Jurkat cells using the protocol described earlier [43] . The treated cells were harvested, washed in PBS and fixed in 70% chilled ethanol for 1 h at room temperature. The cells were washed with PBS, stained with PI by adding PI solution (20 μg ml −1 PI and 0.1 mg ml −1 RNAse A in PBS) for 30 min at 37 °C and subjected to fluorescence-activated cell sorting analysis. VSV-G-pseudotyped pNL4-3-Flag-Tat virus preparation To prepare the VSV-G-pseudotyped Flag-tagged Tat containing HIV-1, 18 μg of pNL4-3 Flag-Tat and 2 μg of VSV-G-expressing plasmid were transfected in a 100-mm cell culture dish of HEK-293T cells using Lipofectamine 2000 (Invitrogen). Medium was replaced with fresh complete DMEM 6 h post transfection. The supernatant containing virus particles were collected 48 h post transfection. The collected virus supernatant was filtered through a 0.45-μm-pore-size filter, and an aliquot was used for p24 assays using β-galactosidase staining of HIV-1 reporter cell line TZM-bl. The viral stock was stored at −80 °C. β-Galactosidase staining of TZM-bl cells The virus-containing medium of J1.1 cells (0.2 ml) of untreated and dicoumarol-treated J1.1 cells was applied to 75% confluent TZM-bl cells in a 12-well plate in presence of 4μg ml −1 Polybrene and incubated for 3 h. Thereafter, the cells were washed twice with DMEM. DMEM with 10% FCS was added and cells were further incubated for 24 h. The infection of HIV-1 in these cells was monitored by β-galactosidase staining as described before [43] . Preparation of Tat supernatant and its application to cells HEK-293T [31] , [44] , [45] , [46] , [47] , [48] , [49] , [50] , [51] , [52] , [53] , [54] cells (10 cm dish) were transfected with 20 μg pCMV-Myc-Tat plasmid with polyethyleneimine and the cells were incubated for 24 h and the supernatant was collected to use it as a source of Tat protein for exogenous application on cells. To observe the effect of dicoumarol on Tat protein, 1 ml supernatant with 1 ml fresh complete DMEM was applied to a 35-mm dish of HEK-293T cells for 4 h for the internalization of Tat protein by these cells. The medium was removed and cells were washed once with DMEM and complete medium was added with or without dicoumarol for further 4 h. Tat protein level was measured by western blotting by Myc antibody. Similarly, the supernatant was applied to Flag NQO1-transfected and untransfected cells and the Tat protein level was measured. Statistical analysis Data obtained were represented as mean±s.e.m. P value was calculated by a two-tailed t -test. Only values of P <0.05 were considered significant. How to cite this article : Lata, S. et al. HIV-1 Rev downregulates Tat expression and viral replication via modulation of NAD(P)H:quinine oxidoreductase 1 (NQO1). Nat. Commun. 6:7244 doi: 10.1038/ncomms8244 (2015).